Mapping of H3N2 influenza antigenic evolution in China reveals a strategy for vaccine strain recommendation One of the primary efforts in influenza vaccine strain recommendation is to monitor through gene sequencing the viral surface protein haemagglutinin (HA) variants that lead to viral antigenic changes. Here we have developed a computational method, denoted as PREDAC, to predict antigenic clusters of influenza A (H3N2) viruses with high accuracy from viral HA sequences. Application of PREDAC to large-scale HA sequence data of H3N2 viruses isolated from diverse regions of Mainland China identified 17 antigenic clusters that have dominated for at least one season between 1968 and 2010. By tracking the dynamics of the dominant antigenic clusters, we not only find that dominant antigenic clusters change more frequently in China than in the United States/Europe, but also characterize the antigenic patterns of seasonal H3N2 viruses within China. Furthermore, we demonstrate that the coupling of large-scale HA sequencing with PREDAC can significantly improve vaccine strain recommendation for China. The seasonal influenza viruses have caused and will continue to cause significant threat to public health, resulting in about three to five million cases of severe illness, and about 250,000–500,000 deaths worldwide each year [1] . At present, massive vaccination is the most effective way to prevent and control the influenza annual epidemics. To achieve effective cross-protection, the antigenicity of a vaccine strain is required to match that of future circulating strains. Unfortunately, the timely and accurate selection of vaccine strains is challenging because the influenza virus changes its antigenicity rapidly by either mutation or reassortment [2] , [3] . As a result, influenza vaccines have to be updated every 2–5 years [4] . To select appropriate strains for vaccine application, the World Health Organization (WHO) has established a network of National Influenza Centers all over the world to monitor the spread and antigenic variation of influenza viruses [5] . Despite this global effort, vaccine recommendation still presents a significant challenge, as evidenced by vaccine mismatches in the past [6] , [7] , [8] , [9] , [10] , [11] . Understanding the antigenic evolution of influenza viruses and their geographical transmission patterns is of critical importance for influenza prevention and control. Studies have indicated that seasonal influenza epidemics are usually seeded from East and Southeast Asia [12] , suggesting that effective seasonal influenza surveillance should focus on these Asian regions. In particular, China has long been thought to have a pivotal role in global influenza transmission because of its temperate climate and diverse geographical features [13] . However, owing to a lack of sufficient viral data, influenza virus antigenic evolution in China and its impact on global influenza dynamics have not been adequately understood. Moreover, reports suggest that vaccine strain selection may be a particular problem in some Asian regions that are sources of new variants [6] , [14] . Given the feasibility of rapid and high-quality sequence determination of HAs or even whole genomes of influenza viruses in influenza surveillance [15] , [16] , development of sequence-based computational approaches has become an indispensable effort to understand the antigenic properties and characteristics of influenza virus evolution. The most widely used method is based on phylogenetic tree analysis of viral HA genes or proteins [17] , [18] . Plotkin et al . [19] used HA protein-sequence clustering to characterize the genetic evolution of the H3N2 virus. We have also reported that nucleotide co-occurrence network across the whole viral genome can capture the general characteristics of influenza antigenic patterns [20] . Recently, several other methods based on sequence information were designed for systematically genetic analysis of influenza virus [21] , [22] , [23] , [24] . These computational works have clearly shown that modeling of the genetic relationships between HA or whole genome sequences of influenza viruses can provide invaluable information for the understanding of their antigenic evolutionary characteristics, holding great promise for rapid influenza surveillance and vaccine strain recommendation. Smith et al . 's [25] clear illustration that antigenic evolution of the H3N2 virus exhibits clusterwise evolutionary patterns, has demonstrated that the antigenic evolution of the H3N2 virus can be viewed as the serial replacement of one antigenic cluster by another [25] , [26] , [27] . Therefore, an optimal vaccine strategy is one that targets an antigenic cluster with a vaccine strain of similar antigenicity. In this study, we introduce PREDAC, a computational approach that uses HA sequences to model the antigenic clusters of H3N2 viruses with high accuracy. The coupling of PREDAC with large-scale HA sequencing of >1,000 H3N2 viruses isolated during 1968–2009 from diverse regions of Mainland China has allowed us to gain a comprehensive picture of the antigenic evolution of H3N2 viruses in China. We further demonstrate that combining PREDAC with large-scale HA sequencing could improve vaccine strain recommendation against seasonal H3N2 viruses for China. PREDAC accurately models the antigenic clusters of H3N2 virus PREDAC models the antigenic clusters of H3N2 viruses based on network representation of the predicted antigenic relationships between viruses ( Fig. 1a ). The antigenic relationship between each pair of viruses in a given group of H3N2 viruses was first predicted based on their HA sequences, and an antigenic correlation network (ACnet) was then constructed by connecting virus pairs predicted to be similar in antigenicity, measured by the log of the odds ratio (that is, the ratio of the predicted likelihood of being antigenically similar to the predicted likelihood of being antigenically distinct). Groups of viruses with similar antigenicity (denoted as predicted antigenic clusters) could then be identified from the ACnet. By using PREDAC, the antigenic evolution of the H3N2 virus can be viewed and analysed in terms of changes in the predicted antigenic clusters. 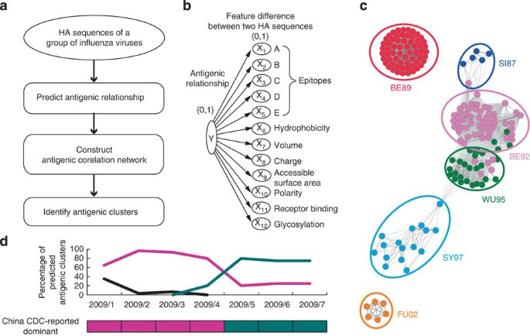Figure 1: Development of PREDAC for modeling the antigenic evolution of the H3N2 virus. (a) The flowchart of PREDAC. (b) The prediction of antigenic relationship by using a feature-based Naive Bayes classifier (feature-based model). This model maps structural and physicochemical features of HA (X1...X12) to antigenic relationships (Y) through naive Bayes theorem. {0, 1} values ofYindicate similar (0) or distinct (1) antigenicity between two viruses. {0, 1} values ofXindicate that discretized features differed between two HAs. (c) Evaluation of the PREDAC in identifying antigenic clusters. In the evaluation, the Smith data25was divided into two parts. One part, which consists of antigenic relationships between the viruses isolated before 1990, was used to develop PREDAC. The other part, which forms five antigenic clusters among the viruses isolated after 1990, was used to evaluate PREDAC. The five known antigenic clusters (named as original clusters from work of Smithet al.25) are colour-coded, and the predicted antigenic clusters with two or more viruses are circled. (d) The use of PREDAC for monitoring the emergence of the recent antigenic cluster PE09 (A/Perth/15/2009-like strains) during 2009. The PE09 antigenic cluster (dark cyan) became predominant in the May of the 2009–2010 season based on our prediction (top panel) and lab confirmation by the China-CDC (bottom panel). Figure 1: Development of PREDAC for modeling the antigenic evolution of the H3N2 virus. ( a ) The flowchart of PREDAC. ( b ) The prediction of antigenic relationship by using a feature-based Naive Bayes classifier (feature-based model). This model maps structural and physicochemical features of HA ( X 1 ... X 12 ) to antigenic relationships ( Y ) through naive Bayes theorem. {0, 1} values of Y indicate similar (0) or distinct (1) antigenicity between two viruses. {0, 1} values of X indicate that discretized features differed between two HAs. ( c ) Evaluation of the PREDAC in identifying antigenic clusters. In the evaluation, the Smith data [25] was divided into two parts. One part, which consists of antigenic relationships between the viruses isolated before 1990, was used to develop PREDAC. The other part, which forms five antigenic clusters among the viruses isolated after 1990, was used to evaluate PREDAC. The five known antigenic clusters (named as original clusters from work of Smith et al . [25] ) are colour-coded, and the predicted antigenic clusters with two or more viruses are circled. ( d ) The use of PREDAC for monitoring the emergence of the recent antigenic cluster PE09 (A/Perth/15/2009-like strains) during 2009. The PE09 antigenic cluster (dark cyan) became predominant in the May of the 2009–2010 season based on our prediction (top panel) and lab confirmation by the China-CDC (bottom panel). Full size image A key element of PREDAC is the accurate prediction of whether two influenza viruses are antigenically similar or distinct (that is, their antigenic relationship) based on their HA sequences. To this end, we devised a machine-learning model using a Naive Bayes classifier to integrate the structural and physicochemical features of HA ( Fig. 1b ). To build this feature-based model, 12 differences in the structural and physiochemical features of each pair of HA sequences were calculated, and a Naive Bayes classifier was then used to integrate these feature differences in order to predict the antigenic relationship between HA sequences. The model was trained using a training data set (Smith data) [25] that consisted of 3,681 antigenically similar HA pairs and 1720 antigenically distinct HA pairs (Methods). In 10-fold cross validations, the feature-based model gave high prediction accuracy: 89.70% and 89.24% for antigenically similar and antigenically distinct pairs, respectively. The performance of PREDAC in predicting antigenic clusters was assessed by the retrospective testing on the Smith data (training on data before 1990 and testing on data after 1990) ( Fig. 1c ). For ease of comparison, each observed antigenic cluster was labeled with a colour, and predicted antigenic clusters with more than one virus were circled. As shown in Fig. 1c , all five known antigenic clusters were identified by PREDAC, and of 174 viruses only 10 viruses were predicted in the wrong clusters. We have further verified the high accuracy of PREDAC in predicting antigenic clusters by testing it on the recent A (H3N2) viruses surveyed in China, for which we will show later. Moreover, to demonstrate whether PREDAC is able to provide real-time and accurate monitoring of the emergence of antigenic clusters, we monitored the development of a recent antigenic cluster PE09 (A/Perth/15/2009-like strains) by applying PREDAC to the large-scale HA sequences determined during influenza surveillance by the Chinese Center for Disease Control and Prevention (China CDC). PREDAC detected its predominance in May 2009 ( Fig. 1d ). To test whether our computational detection is both timely and accurate, we used the haemagglutination inhibition (HI) assay to determine the antigenic properties of 54 viruses isolated between March and August, 2009 ( Supplementary Table S1 ). The HI assay showed that ∼ 90% of the predicted antigenic variants isolated after May 2009 were indeed antigenically different from the vaccine strain of the last predicted antigenic cluster (≥fourfold titer), and ∼ 71% of the viruses isolated in March and April did not change their antigenicity ( Large-scale sequencing and analysis of H3N2 HAs in China For a better understanding of the antigenic evolution and transmission of H3N2 viruses in China, we carried out large-scale sequencing of HA from 1,071 H3N2 viruses isolated between 1968 and 2009 from a variety of representative regions in Mainland China ( Supplementary Data 1 ). 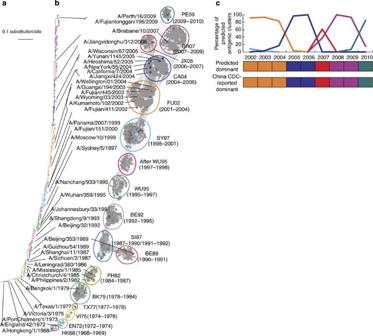Figure 2: Characterization of the antigenic evolution of the H3N2 virus in China. (a) Phylogenetic tree of HA1 protein sequences of 1,438 viral isolates from Mainland China (additional vaccine strains were included). (b) Predicted ACnet and antigenic clusters for the 1,438 viruses from Mainland China (additional vaccine strains were included). The predicted antigenic clusters are coloured and named according to the vaccine strains (location in the tree and network are directed by the line) contained in the clusters. The time of dominance for each cluster is given in parentheses. (c) Validation of the predicted antigenic clusters for viruses isolated from 2002–2010. The dynamic changes in the percentage of antigenic clusters were recorded on a monthly basis for recent clusters. The bottom two panels show the distributions of predicted dominant antigenic clusters and the actual dominant antigenic strains reported by the China CDC in each influenza season between 2001–2002 and 2009–2010. A dominant cluster was defined as one in which >50% of the viruses were present. Figure 2a shows a phylogenetic tree for 1,438 H3N2 viruses isolated in Mainland China (including 367 viruses whose HA sequences were determined previously). Although phylogenetic analysis has been widely used to understand the genetic evolution of the influenza virus, using the method to delineate the virus antigenic evolution is not straight forward [25] . We applied PREDAC to construct an ACnet and predict antigenic clusters for the 1,438 H3N2 viruses ( Fig. 2b ). In total, 20 antigenic clusters were identified, 17 of which were considered as dominant antigenic clusters as each of them included >50% of the viruses in at least one season ( Fig. 2b , Supplementary Table S2 ). The 17 predominant antigenic clusters included ∼ 99% of the viruses, and each of the clusters persisted for one to five seasons ( Fig. 2b ). Figure 2: Characterization of the antigenic evolution of the H3N2 virus in China. ( a ) Phylogenetic tree of HA1 protein sequences of 1,438 viral isolates from Mainland China (additional vaccine strains were included). ( b ) Predicted ACnet and antigenic clusters for the 1,438 viruses from Mainland China (additional vaccine strains were included). The predicted antigenic clusters are coloured and named according to the vaccine strains (location in the tree and network are directed by the line) contained in the clusters. The time of dominance for each cluster is given in parentheses. ( c ) Validation of the predicted antigenic clusters for viruses isolated from 2002–2010. The dynamic changes in the percentage of antigenic clusters were recorded on a monthly basis for recent clusters. The bottom two panels show the distributions of predicted dominant antigenic clusters and the actual dominant antigenic strains reported by the China CDC in each influenza season between 2001–2002 and 2009–2010. A dominant cluster was defined as one in which >50% of the viruses were present. Full size image Predicted antigenic clusters capture H3N2 evolution in China We further evaluated whether the predicted antigenic clusters accurately describe the actual antigenic patterns of the H3N2 virus in China. When the vaccine strains recommended by WHO and other candidate vaccine strains characterized by China CDC were included in the modeling, we found that all the antigenically distinct vaccine strains and candidate vaccine strains were separated into different predicted antigenic clusters ( Fig. 2b and Supplementary Table S2 , additional vaccine strains were included). Moreover, most of the H3N2 viruses isolated in China tended to cluster with these vaccine strains. Notably, of the 17 predicted predominant antigenic clusters, 16 contained vaccine strains and candidate vaccine strains of similar antigenicity. The accurate assignment of vaccine strains to the predicted antigenic clusters indicates the effectiveness of PREDAC in modeling the antigenic evolution of H3N2 viruses in China. When comparing with the China CDC-monitored antigenic data for the H3N2 viruses circulated from 2002 to 2009 using HI assays, we obtained an even closer fit between the observed and predicted antigenic clusters, further validating our approach. According to the China CDC surveillance results, the H3N2 viruses circulated from 2001–2002 to 2009–2010 seasons formed five groups with distinct antigenicity ( Fig. 2c ). For these viruses, PREDAC also predicted five antigenic clusters that matched those characterized by the China CDC ( Fig. 2c ). The above tests demonstrate that PREDAC-predicted antigenic patterns accurately capture the antigenic evolution of H3N2 viruses in China. Comparative analysis of predicted antigenic clusters As shown in Fig. 2b , the predicted ACnet and antigenic clusters vividly depict the antigenic patterns of H3N2 viruses in China. Interestingly, the changes of the predicted antigenic clusters follow a trunk-like pattern; most of the antigenic clusters are located on the main trunk. However, we observed two branches off the trunk: one contains A/Beijing/353/1989-like strains (BE89) and the other contains A/Jiangxidonghu/312/2006-like strains (JX06). A close examination of the two branches further reveals the special patterns of local dominance of H3N2 virus in China and their impacts on the global transmission. The BE89 was first detected in China and was suggested as vaccine strain by WHO, but it was unable to replace the old antigenic cluster A/Sichuan/1/1987-like viruses (SI87) in China. However, in Europe and North America, the BE89 indeed displaced SI87 and became dominant during 1990–1991 ( Fig. 3 ). Interestingly, JX06 was also first detected and became dominant in China during 2006–2007, but it did not get chance to become dominant in Europe and the USA ( Fig. 3 ). 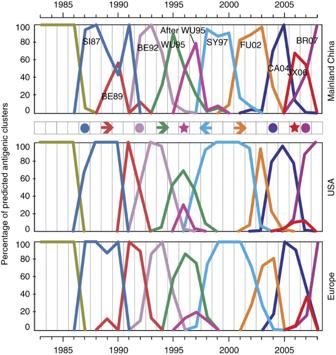Figure 3: Comparison of antigenic patterns of H3N2 viruses between different regions during 1983–2008. Dynamic changes in the percentage of antigenic clusters were recorded on a yearly basis for China, the United States and Europe. For comparison, only the predicted dominant antigenic clusters that contain >50% of the viral isolates in at least 1 year in any of the three regions were considered. The emergence time of a novel predicted dominant antigenic cluster in a location was defined as the earliest year when the cluster contained at least one quarter (25%) of the viral isolates in the location. Symbols represent the predicted dominant antigenic clusters unique to China (star), the earlier (right-pointing arrow), or later (left-pointing arrow) emergence of predicted dominant antigenic clusters in China than the United States and Europe, and the emergence time of predicted dominant antigenic clusters being the same in all three regions (dot). Figure 3: Comparison of antigenic patterns of H3N2 viruses between different regions during 1983–2008. Dynamic changes in the percentage of antigenic clusters were recorded on a yearly basis for China, the United States and Europe. For comparison, only the predicted dominant antigenic clusters that contain >50% of the viral isolates in at least 1 year in any of the three regions were considered. The emergence time of a novel predicted dominant antigenic cluster in a location was defined as the earliest year when the cluster contained at least one quarter (25%) of the viral isolates in the location. Symbols represent the predicted dominant antigenic clusters unique to China (star), the earlier (right-pointing arrow), or later (left-pointing arrow) emergence of predicted dominant antigenic clusters in China than the United States and Europe, and the emergence time of predicted dominant antigenic clusters being the same in all three regions (dot). Full size image To better understand the dynamic changes in influenza antigenic patterns in China and their impact on global transmission, PREDAC was applied to model the antigenic evolution of 9,386 H3N2 viruses collected from all over the world during 1968–2009 (including 1,071 newly sequenced viruses from China). For comparison, we tracked dynamic changes in predicted antigenic clusters in China, the United States and Europe during 1983–2008 ( Fig. 3 ), a period when there was sufficient viral data for these regions. As seen in Fig. 3 , of the 10 predicted antigenic clusters that were predominant in at least one season during the past >20 years, 10 such antigenic clusters were observed in China, only one cluster emerged later than those identified in the United States or Europe (left-pointing arrow), the remaining nine clusters being either only predominant in China (two clusters marked by stars), emerging earlier than those identified in the United States or Europe (three clusters, right-pointing arrows) or emerging at the same time (four clusters marked by dots). To generate stronger statistics and avoid sampling bias with respect to region and time, we performed a simulation by randomly choosing 10 sequences from each location (China/the United States) in each year. The simulation was performed 1,000 times. We found that in 70% of the simulated cases, China is more likely to have more dominant antigenic clusters than the United States. Moreover, for novel antigenic clusters, in 95% of the simulated cases they are more likely to emerge first in China than in the United States. The observation that China is more likely to lead global influenza transmission than the the United States or Europe was even more evident ( Supplementary Fig. S1 ), when we made a fine month-by-month comparison based on recent influenza seasons during 2002–2008, a period for which we were able to obtain sufficient monthly information. Of the four predicted antigenic clusters, FU02 (A/Fujian/411/2002-like strains), CA04 (A/California/7/2004-like strains), JX06 and BR07 (A/Brisbane/10/2007-like strains), three (FU02, CA04 and JX06) were clearly more advanced in China. Notably, when we looked at the dynamics of antigenic patterns within China by dividing it into Northern China (temperate regions) and Southern China (tropical regions) according to Qin Mountain and Huai River ( Supplementary Data 1 ), we found that new antigenic variants are more likely to emerge first in Tropical China and then transmitted to Temperate China ( Supplementary Fig. S2 ), although such difference has not been observed between Coastal China and Mainland China ( Supplementary Fig. S3 ). PREDAC improves vaccine strain recommendation for China The greater antigenic diversity and leading role in global influenza transmission could confound flu control efforts in China. Here, we would like to ask whether the coupling of large-scale HA sequencing with PREDAC during influenza surveillance could improve vaccine strain recommendation for China. 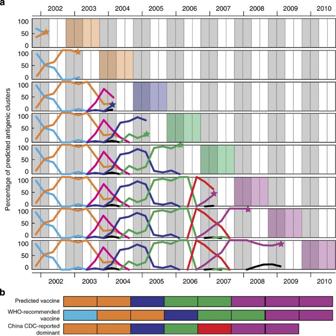Figure 4: Automatic vaccine strain recommendations based on the H3N2 viruses monitored in China. (a) Season by season vaccine strain recommendations for the influenza seasons from 2002–2003 to 2009–2010 based on the H3N2 viruses monitored in China before March 15 of each year from 2002–2009. Dynamic changes in predicted antigenic clusters were monitored by quarter. For clarity, the antigenic clusters prior to 2002 are not shown. Asterisks indicate the dates (March 15 in this case) for vaccine strain recommendation. Gray backgrounds indicate winter seasons in the Northern Hemisphere. The coloured backgrounds indicate the season in which the predicted vaccine strains were to be used. Different coloured lines represent different clusters. (b) A comparison of the predicted and WHO-recommended vaccine strains for targeting dominant strains in China. Colours used represent clusters as in (a). Vaccine strains recommended by WHO (WHO-recommended vaccine) were extracted from the WHO website55,56,57,58,59,60. Figure 4a illustrates the procedure of vaccine recommendations made on March 15 using a threshold percentage of 15% by modeling the dynamic changes in predicted antigenic clusters of H3N2 viruses in China during 2002–2009. Figure 4: Automatic vaccine strain recommendations based on the H3N2 viruses monitored in China. ( a ) Season by season vaccine strain recommendations for the influenza seasons from 2002–2003 to 2009–2010 based on the H3N2 viruses monitored in China before March 15 of each year from 2002–2009. Dynamic changes in predicted antigenic clusters were monitored by quarter. For clarity, the antigenic clusters prior to 2002 are not shown. Asterisks indicate the dates (March 15 in this case) for vaccine strain recommendation. Gray backgrounds indicate winter seasons in the Northern Hemisphere. The coloured backgrounds indicate the season in which the predicted vaccine strains were to be used. Different coloured lines represent different clusters. ( b ) A comparison of the predicted and WHO-recommended vaccine strains for targeting dominant strains in China. Colours used represent clusters as in ( a ). Vaccine strains recommended by WHO (WHO-recommended vaccine) were extracted from the WHO website [55] , [56] , [57] , [58] , [59] , [60] . Full size image For better vaccine strain recommendation, we investigated how key parameters of the program affect the efficiency of vaccine strain prediction ( Supplementary Methods ). Table 1 summarizes how the two key parameters, namely threshold percentage and prediction date, affect vaccine strain predictions for China for the seven influenza seasons from 2002–2009. As shown in Table 1 , the appropriate choice of parameter combinations can lead to the best possible protection of H3N2 virus in China. Notably, when we chose to recommend vaccine strains in mid-March (1 month later than the mid-February date used by the WHO), six of the seven predicted vaccine strains matched the actual circulating strains in China (comparing panels 1 and 3 of Fig. 4b ), significantly better than the WHO-recommended vaccine strains, which had only two matches for China (comparing panels 2 and 3 of Fig. 4b ). Table 1 Numbers of correctly predicted vaccine strains for China during the seven seasons from 2002–2003 to 2008–2009. Full size table In this study, through development of an effective computational framework coupled with determination of HA sequences of >1,000 H3N2 viruses isolated during 1968–2009 from diverse regions of Mainland China, we have not only mapped the antigenic evolution of H3N2 viruses in China, but also proposed an effective influenza surveillance program for flu planning in China. Timely and accurate recommendation of vaccine strains is critical for influenza prevention and control. Despite the global efforts, the current vaccine strain recommendation strategy has caused significant lags for China (comparing panels 2 and 3 of Fig. 4b ). As indicated by our study, the prediction lags for China could be partly because of the lack of sufficient data for vaccine strain decision and partly because of the rapid decline and rise of strains after vaccine strain recommendations ( Fig. 3 ). Therefore, how to implement an effective seasonal influenza-monitoring program in China is critical for its vaccine strain recommendation. Owing to the rapid development of sequencing technology, DNA sequencing is becoming cheaper and faster, which can make the sequence data available even in a couple of days. Moreover, compared with HI data, sequence data is very reliable and will not vary from one lab to another. Large-scale sequencing is now widely used in influenza surveillance [28] , [29] . To accompany the large-scale sequencing effort in influenza surveillance, our work has further developed a sequence-based program for effective antigenicity inference. We demonstrated that the informatics framework PREDAC we developed can effectively infer antigenic clusters from HA sequences, and thus can provide a very important tool in the influenza surveillance and vaccine strain recommendation when coupled with large-scale HA sequencing. Previously, many computational approaches were designed to either predict antigenic variants [18] , [30] , [31] , [32] , [33] , [34] , [35] , [36] or to model evolutionary patterns for the H3N2 virus [19] , [20] , [21] , [23] , [24] . In our study, the prediction of antigenic variants and the modeling of antigenic evolutionary patterns are integrated into one computational framework, PREDAC. In developing models for predicting antigenic relationships, previous efforts mainly relied on changes in specific amino acids at certain residues that have been observed in the evolution of influenza virus HA (called site-dependent models). Our work, however, directly considers 12 structural and physicochemical features of HA that are reported to or are thought to affect the antigenic properties of influenza HA. We have demonstrated that our feature-based model can predict antigenic relationships with high accuracy (the contributions of individual features are given in Supplementary Table S3 ). The feature-based model is a more generalized model that does not rely on specific amino-acid changes, and is thus able to model antigenic changes due to new amino-acid changes. Moreover, by integrating the highly accurate prediction of antigenic relationships into a network model, the computational approach developed here, PREDAC, is reliable for modeling influenza antigenic patterns. We have demonstrated the effectiveness of PREDAC in modeling the antigenic clusters for the viruses isolated from Mainland China, which accurately matched the antigenic patterns observed by China CDC ( Figs 1d and 2c ). As a machine learning-based method, PREDAC could be further improved by using more representative and accurate antigenic data during training and by incorporating other relevant features underlying HA-antibody interactions. As PREDAC is a generalized model, it can be easily applied to the other two seasonal viruses with proper modification. For its critical role in global influenza transmission, many analysts have put China under the spotlight. However, because of a lack of systematic analysis, much remains unclear regarding what the antigenic patterns are in China and how they affect global influenza transmission. The comprehensive picture of the influenza antigenic evolution in China has enabled us to explore the detailed antigenic evolution patterns in China and their impact on global influenza transmission, which has significantly deepened the understanding of the dynamics and complexity in global influenza transmission. Our systematic work has not only revealed a greater antigenic diversity in China but also shown a significant difference in the time and magnitude of emergence of antigenic clusters between China and the United States/Europe. This complicates the global influenza prevention and control, underscoring the necessity and importance of development of effective local influenza planning strategies for the source regions. For example, the vaccine strain we predicted for the 2002–2003 influenza season based on China data targeted Fujian-like viruses. The Fujian antigenic cluster (FU02) indeed became dominant in China in the 2002–2003 influenza season ( Figs 2c and 3 ); however it did not dominate in the United States/Europe until at least one influenza season later [37] , [38] ( Fig. 3 ). The local dominance of some antigenic clusters also adds uncertainty to global vaccination planning. For example, the JX06 antigenic cluster was predominant in China during 2006–2007 season, but it did not dominate in the United States and Europe ( Fig. 3 ). Recently Bahl et al . [39] also showed that the seasonal H3N2 epidemics are geographically and temporally structured, suggesting localized annual epidemics. Therefore, in an effort to coordinate the global vaccine strategy, local planning of influenza prevention and control is critical [40] , [41] . Moreover, if an influenza variant can be contained locally, particularly where it emerges, this should benefit the rest of the world. HA sequence data and sequence analysis Large-scale HA sequencing of 1,071 H3N2 viruses sampled from diverse and representative regions of Mainland China between 1968 and 2009 were carried out by the China CDC (366 from Northern China/Temperate region and 705 from Southern China/Tropical region, see Supplementary Data 1 for details). Other sequence data were downloaded from the National Center for Biotechnology Information Influenza Virus Resource [16] ( http://www.ncbi.nlm.nih.gov/genome/FLU/FLU.html ). All HA1 sequences were aligned with ClustalW [42] . A phylogenetic tree for the viruses isolated in China was constructed using PhyML [43] version 2.4.5, with A/Beijing/1/1968 as the root. Detailed information regarding HA sequence data and sequence analysis is described in the Supplementary Methods . A feature-based model for antigenic relationship prediction To predict whether two viruses are antigenically similar or distinct (that is, their antigenic relationship), we developed a machine-learning approach ( Fig. 1b ). The development of the method involves five steps described as follows: We constructed a training data set. Recently, Smith et al . [25] systematically characterized the antigenic relationships between 253 viruses isolated between 1968 and 2003 using a HI assay, and grouped these viruses into 11 antigenic clusters through data modeling. We refer to pairs of strains from the same antigenic cluster as antigenically similar pairs, and pairs of strains from different antigenic clusters are referred to as antigenically distinct pairs. Totally, there are 4,849 antigenically similar and 27,029 antigenically distinct pairs. In order to balance our training data set, also considering that 99% pairs with more than nine mutations are antigenic distinct pairs, we only consider pairs with no more than nine mutations as our training data set, which include 3,681 antigenic similar pairs and 1,720 antigenic distinct pairs. We selected features that contribute to influenza antigenic changes. We considered 12 structural and physicochemical properties or features that have been reported to or are thought to affect the antigenic properties of influenza HA. These 12 features include five known H3N2 virus HA epitopes, five physicochemical properties of amino acids (hydrophobicity, volume, charge, polarity and accessible surface area), receptor binding and glycosylation, which can be further classified into three groups. Group I includes the five known HA epitopes from the A (H3N2) virus [44] , as it is widely recognized that the extent of antigenic changes correlates with the number of mutations within these epitopes [45] . Group II includes the basic physicochemical properties of surface amino-acid residues that are thought to affect antigen–antibody interactions [46] . These physicochemical properties include hydrophobicity, volume, charge, polarity and accessible surface area of the amino acids. Group III includes the amino acids that are associated with receptor binding and glycosylation. As it has been recognized that influenza virus antigenic change is closely related to its receptor binding, and that glycosylation on HA can mask antigenic sites and help the flu virus to evade host immune surveillance [47] , [48] , the amino-acid changes associated with receptor binding and glycosylation has important roles in the antigenic evolution of influenza virus. We measured the differences in the 12 features between HA pairs. For feature j ( j =1, ..., 12), its score for a given HA pair i ( i = 1, ..., N . N is the total number of HA pairs in the training data is denoted as s ij , and is computed as follows: when j refers to one of the five known epitopes, s ij is calculated as the number of amino-acid differences between i ; when j refers to one of the five physicochemical properties, s ij is calculated as the average change in quantitative values of j between i . The quantitative values of the five physicochemical properties for the 20 amino acids were obtained from the Amino Acid index database [49] (the database entries FASG890101, GRAR740103, ZIMJ680104, CHAM820101 and JANJ780101 recorded quantitative descriptions of hydrophobicity, volume, charge, polarity and accessible surface area of the 20 amino acids, respectively). If the number of sites with amino-acid changes was greater than three, only the top three sites with maximal changes were considered in the calculation of s ij . When j refers to glycosylation, s ij is calculated as the number of changed glycosylation sites as predicted using NetNGlyc [50] (the predicted glycosylation sites change about 0.1 site per year). When j refers to receptor binding, s ij is calculated as the average of the shortest Euclidean distances between the sites with amino-acid changes and the three structure elements (130-loop, 190-helix and 220-loop) of the receptor-binding region [51] . The Euclidean distance between two residues was calculated between their respective C-α atoms. To calculate the shortest Euclidean distance of a mutated residue to the receptor-binding region, we first computed its Euclidean distances to all residues located in the three structure elements using the structure of A/Aichi/2/1968 as template (pdb 1HGF) [52] , and then the shortest Euclidean distance was used in our study. If more than three mutations occurred, only the top three shortest Euclidean distances were considered in the calculation of s ij . On the basis of the above calculations, an HA pair i in the training data set can be represented by a vector ( s ij ), j =1, ..., m ; m =12. Thus, given a training data set consisting of N ( N =5,401 for Smith data) pairs of HA sequences with known antigenic relationships (denoted as y =( y i ), i =1, ..., N : y i =0 represents antigenic similarity and y i =1 for differences in antigenicity), a score matrix S =( s ij ) N × m can be used to represent feature values for all HA pairs in the training data set. We discretized each feature to avoid overfitting. Each feature was discretized using the method proposed by Yuan et al [53] . In brief, a threshold cut-off for the continuous scores s ij corresponding to a feature is chosen so as to best distinguish the antigenic relationship in given training data set (the discretization cut-off values for the 12 features have been provided in Supplementary Table S4 ). The purpose of this process is to avoid overfitting by assigning only two values (0 or 1) to each feature [53] . Accordingly, the score matrix S becomes a 0–1 matrix, and it is denoted as X =( x ij ), i =1, ..., N ; j =1, ... m . Finally, we built a Naive Bayes classifier to predict antigenic relationships. The Naive Bayes classifier is a statistical learning method which has been widely used for classification problems in biology. For a given pair of strains, the values for the 12-feature variables X j ( j =1, ... m ) can be calculated based on their sequences. To predict the antigenic relationship Y (0, 1 represent antigenic similarity and differences in antigenicity, respectively) for the given pair of strains, we used the Bayes theorem: The odds ratio was used to denote the extent of antigenic similarity, and is computed as: Given a training data set that consists of label vector y =( y i , ..., y N ) and descretized score matrix X =( x ij ), i =1, ..., N ; j =1, ... m , the probabilities on the left side of equation (2) were derived by following Yuan et al . 's [54] method: Based on these probabilities determined using the training data set, the odds ratio can be easily calculated according to equation (2). If the odds ratio is >1, the antigenic relationship of the two viruses is regarded as antigenically similar, otherwise as antigenically distinct. The greater the odds ratio is, the more likely it is that the two viruses are antigenically similar. The model performance was assessed using cross validation and retrospective testing on the training data (details see Supplementary Methods ). Development of PREDAC for analysis of antigenic evolution The PREDAC includes the following three steps ( Fig. 1a ). In step 1, for a group of viruses of interest, the antigenic relationships between there HA sequences were predicted using the feature-based model described above. Then in step 2, all viral pairs predicted to be antigenically similar (odds ratio >1) were connected to generate ACnet. In step 3, to infer antigenic clusters, viruses from the ACnet with similar antigenicity were grouped using the MCL program [54] , which is designed for network clustering. Details regarding how to use MCL to identify antigenic clusters see Supplementary Methods . PREDAC-based vaccine strain recommendation program To recommend a vaccine strain based on a large-scale HA sequencing of H3N2 virus surveyed at different time points, we applied PREDAC to construct ACnets and further identify antigenic clusters for the viruses isolated from 1995 to the given date. Dynamic changes for the antigenic clusters were visualized as changes in the percentages of viral isolates belonging to an antigenic cluster each quarter. At the time of vaccine strain recommendation (for example, March 15 in Fig. 4a ), if a new cluster emerges with a percentage over a certain threshold, called threshold percentage (15% for example in Fig. 4a ), it is predicted to become dominant in the upcoming season. If two or more novel antigenic clusters exceeded the given threshold, the one with the highest percentage was considered. Therefore, the vaccine strain for the upcoming season needs to be updated. For example, as shown in Fig 4a , the novel antigenic clusters detected with a percentage of >15% by time of March 15 in 2002 (marked by brown), 2004 (blue), 2005 (green) and 2007 (scarlet) were recommended as vaccine strains for the winter seasons 2002–2003, 2004–2005, 2005–2006 and 2007–2008, respectively. Otherwise, it was assumed that the antigenic cluster that dominated in the previous season would continue to dominate in the coming season, and it was not necessary to update the vaccine strain. Accession codes: The sequence data have been uploaded to the Genbank database under accession code CY107862 to CY108409 , CY109411 to CY108435 , CY108437 to CY108934 . How to cite this article: Du, X. et al . Mapping of H3N2 influenza antigenic evolution in China reveals a strategy for vaccine strain recommendation. Nat. Commun. 3:709 doi: 10.1038/ncomms1710 (2012).